Phylogenetic measures of biodiversity and neo- and paleo-endemism in AustralianAcacia Understanding spatial patterns of biodiversity is critical for conservation planning, particularly given rapid habitat loss and human-induced climatic change. Diversity and endemism are typically assessed by comparing species ranges across regions. However, investigation of patterns of species diversity alone misses out on the full richness of patterns that can be inferred using a phylogenetic approach. Here, using Australian Acacia as an example, we show that the application of phylogenetic methods, particularly two new measures, relative phylogenetic diversity and relative phylogenetic endemism, greatly enhances our knowledge of biodiversity across both space and time. We found that areas of high species richness and species endemism are not necessarily areas of high phylogenetic diversity or phylogenetic endemism. We propose a new method called categorical analysis of neo- and paleo-endemism (CANAPE) that allows, for the first time, a clear, quantitative distinction between centres of neo- and paleo-endemism, useful to the conservation decision-making process. Biodiversity is not just species—instead it is the full set of nested clades representing phylogenetic relationships among organisms at all levels. Species are, at best, only one level of clades among thousands, smaller and larger [1] . Unfortunately, biodiversity is most often studied solely at the species level, which misses both the full richness of patterns that can be inferred from the full tree of life, and the analytical power that comes from a phylogenetic approach. Our perception of biodiversity patterns becomes more complete when phylogenetic methods are added to traditional species-based methods [2] , [3] . Likewise, endemism is not just about species, even though virtually all endemism studies focus solely at the species level. Clades at all levels can be endemic and all levels are relevant to discovery and evaluation of centres of endemism. Endemism, rather than being species-centric, should be more broadly defined to mean ‘the geographic rarity of that portion of a phylogenetic tree found in a given area’. This phylogenetically based definition encompasses clades that are at the traditional species level, but also takes into account clades larger than or smaller than named species, and so provides a more complete picture of endemism. The relevance of phylogeny to ecology and evolution is widely recognized and has revolutionized those fields [4] , [5] , [6] , [7] , [8] ; however, the relevance of phylogeny to biodiversity assessment and conservation remains generally underappreciated despite groundbreaking steps in this direction [9] , [10] . Phylogenetic measures of biodiversity were pioneered by Faith [11] , who developed the concept of phylogenetic diversity (PD), which has been increasingly explored in recent years [12] , [13] , [14] , [15] . Faith et al. [12] and Rosauer et al. [16] then established phylogenetic concepts of endemism. Faith et al. ’s approach was to identify what parts of a phylogenetic tree are absolutely restricted to a given region, an approach that could be called ‘absolute phylogenetic endemism’. Rosauer et al. ’s approach considered the relative breadth of geographic distribution of parts of a phylogenetic tree that are found in a given region, an approach that could be called ‘weighted phylogenetic endemism’. Rosauer et al. ’s definition (which is applied throughout this paper and referred to as PE) is directly analogous to weighted endemism for species (or other terminal taxa in a phylogeny, abbreviated WE [17] ). The range of either a branch or species can be measured using various units, for example, the number of grid cells it occurs in, and the range of a branch is the union of ranges of terminal taxa descended from it. PE for a region is the length of a branch multiplied by the proportion of its range which occurs in that region (the inverse of the range for a single-cell case), summed over all the branches found in that region, just as species endemism (WE) for a region is one multiplied by the proportion of a species’ range which occurs in that region, summed over all species in the region [16] . It has long been recognized that there are two kinds of endemic species: neo-endemics—recently diverged species that are endemic because of lack of dispersal/migration out of their ancestral area; and paleo-endemics—old species that were perhaps more widespread in the past and are now restricted to a local region [18] , [19] , [20] . This traditional taxonomic formulation is suboptimal for two reasons. The first is theoretical: this formulation only deals with species, yet clades at all levels can be endemic. The second is methodological: a rigorous analytical approach has so far been lacking to separate the two kinds of endemism in practice. This paper aims to solve both issues by presenting and illustrating a general approach to studying endemism at all phylogenetic scales. It provides the first quantitative measure to clearly distinguish centres of neo-endemism from centres of paleo-endemism. Our approach also allows the discovery of areas that are centres of both neo- and paleo-endemism, we call such areas ‘centres of mixed-endemism’, while centres with extremely high values of both we call ‘centres of super-endemism’. Another important step forward was the development of methods to examine differences among regions in PD: ‘PD-dissimilarity’ [21] or ‘phylogenetic beta-diversity’ [22] , and to apply these to conservation concerns, for example, ‘PD-complementarity’ [12] . These methods use a pairwise distance matrix among regions as a basis for cluster analyses and ordinations, but instead of standard distance metrics based on the proportion of shared species, they use a phylogenetically based metric on the basis of the proportion of shared branches. Australia presents the best current opportunity for studying large-scale patterns of PD and PE in plants because of the nearly complete digitization of herbarium collections by Australia’s Virtual Herbarium ( http://avh.ala.org.au/ ). Here we take advantage of this rich source of distributional data, and the generation of new DNA sequence data gathered for phylogenetic purposes, to study one of the most diverse clades of Australian plants, the legume genus Acacia . Over 1,000 species have been described within the clade of Australian Acacia [23] , <1% of which occur beyond Australia [24] . It is estimated that this clade diverged from its closest relatives around 25 Myr ago and has spread into most Australian climatic areas including the monsoonal tropics, the arid interior and the Mediterranean climates of southern Australia [24] . Acacia has diversified into a vast array of vegetative forms during this radiation and this has resulted in a complicated morphologically based taxonomic classification [25] . Basic patterns of species richness (SR) and endemism in Acacia across the Australian continent are known [26] ; however, little is known about the spatial distribution of Acacia in a phylogenetic context. Our goals were to: (1) map patterns of PD and PE in Acacia across the Australian continent; (2) explore properties of a new index (relative phylogenetic diversity or RPD), designed to identify and distinguish areas of phylogenetic overdispersion and clumping that reflect signals of biogeographic history and ecological processes; (3) explore properties of another new index (relative phylogenetic endemism or RPE), within a novel framework called Categorical Analysis of Neo- And Paleo-Endemism (CANAPE), designed to identify and distinguish centres of neo-endemism from centres of paleo-endemism in a rigorous way; (4) develop novel hypothesis tests for these measures using appropriate null models; (5) examine similarities and differences among the identified centres of PE with respect to implications for conservation. We found that, while SR and PD are generally correlated, there are regions with much more PD or much less PD than expected given our hypothesis test. The new RPD index works well to distinguish these regions and gives insight into ecological and biogeographic processes. Likewise, while WE and PE are generally correlated, there are regions with much more PE or much less PE than expected given our two-step CANAPE hypothesis test using the new RPE index, corresponding to centres of paleo-endemism and neo-endemism, respectively. When comparing the discovered centres of endemism using a phylogenetic beta-diversity analysis, we found interesting biogeographic patterns of similarity in the parts of the phylogenetic tree shared among areas, and were able to identify areas of particular conservation concern where parts of the phylogeny remain unprotected. Phylogenetic analyses The final molecular data set had 4,044 aligned nucleotides across six loci. The maximum likelihood tree topology recovered is shown in Supplementary Fig. 1 and the data set and tree are lodged in TreeBase (ID 13659, http://treebase.org/treebase-web/search/study/summary.html?id=13659 ). Basic biodiversity analyses Maps of SR, WE, PD and PE are shown in Fig. 1 . Bivariate plots and linear regression analysis examining the relationships among these variables revealed that they are significantly positively correlated, but with variable scatter. For example, while PD is significantly related to SR, there is still reasonable scatter ( r 2 =0.876; Supplementary Fig. 2 ), and no sign of a plateau at the highest levels of richness found in this study (at very high richness, a decline in increase of PD would be expected as most of the tree becomes represented). PE is also significantly, but less closely, related to SR ( r 2 =0.400; Supplementary Fig. 3 ). PD is significantly related to PE, but again with much scatter ( r 2 =0.475; Supplementary Fig. 4 ). 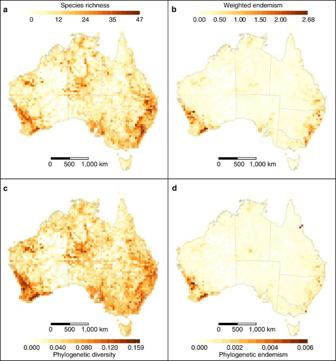Figure 1: Maps showing basic biodiversity patterns in AustralianAcacia. (a) SR; (b) WE; (c) PD; and (d) PE. Figure 1: Maps showing basic biodiversity patterns in Australian Acacia . ( a ) SR; ( b ) WE; ( c ) PD; and ( d ) PE. Full size image Development of null hypotheses It is important to look at the expected values of these variables in light of appropriate null hypotheses, thus we developed two new metrics: RPD and RPE as the basis for null hypotheses to be tested statistically using a randomization approach (see Methods for details about these two derived metrics and the hypothesis test). Randomization tests Randomization-based significance tests of PD, RPD, PE and RPE are shown in Fig. 2 . Areas of significantly high PD include southwestern Australia, Tasmania and the southern coast of South Australia; areas of significantly low PD are scattered broadly across most of the remainder of the continent ( Fig. 2a ). Areas of significantly high RPD include southwestern Australia, central Australia and the southern coast of South Australia, with a few cases in northern and eastern Australia; areas of significantly low RPD include many locations in the eastern Great Dividing Range and southeastern Australia ( Fig. 2b ). Areas of significantly high PE include southwestern and western Australia and scattered areas along the east coast and Tasmania; areas of significantly low PE are scattered broadly across the interior of the continent ( Fig. 2c ). Areas of significantly high RPE include southwestern Australia, the Pilbara Region, central Australia, wet tropic sites in Queensland and Tasmania, while areas of significantly low RPE are mostly found in the southeast part of the continent; interestingly the northern region of the Monsoonal tropics is underrepresented for both ( Fig. 2d ). 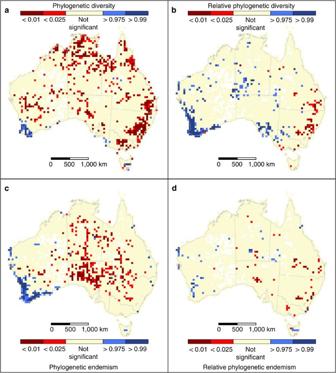Figure 2: Maps showing significance levels resulting from of a randomization test in AustralianAcacia. White cells contain no records; beige cells are not significant. (a) PD: the red values indicate grid cells that contain significantly less PD than expected; the blue values indicate grid cells that contain significantly more PD than expected. (b) RPD: the red values indicate grid cells that contain significantly less RPD than expected; the species present in that cell are significantly more closely related than expected. The blue values indicate grid cells that contain significantly more RPD than expected; the species present in that cell are significantly more distantly related than expected. (c) Phylogenetic endemism (PE). The red values indicate grid cells that contain significantly less PE than expected; the blue values indicate grid cells that contain significantly more PE than expected. (d) Relative phylogenetic endemism (RPE). The red values indicate grid cells that contain significantly lower RPE than expected; the blue values indicate grid cells that contain significantly higher RPE than expected. Figure 2: Maps showing significance levels resulting from of a randomization test in Australian Acacia. White cells contain no records; beige cells are not significant. ( a ) PD: the red values indicate grid cells that contain significantly less PD than expected; the blue values indicate grid cells that contain significantly more PD than expected. ( b ) RPD: the red values indicate grid cells that contain significantly less RPD than expected; the species present in that cell are significantly more closely related than expected. The blue values indicate grid cells that contain significantly more RPD than expected; the species present in that cell are significantly more distantly related than expected. ( c ) Phylogenetic endemism (PE). The red values indicate grid cells that contain significantly less PE than expected; the blue values indicate grid cells that contain significantly more PE than expected. ( d ) Relative phylogenetic endemism (RPE). The red values indicate grid cells that contain significantly lower RPE than expected; the blue values indicate grid cells that contain significantly higher RPE than expected. 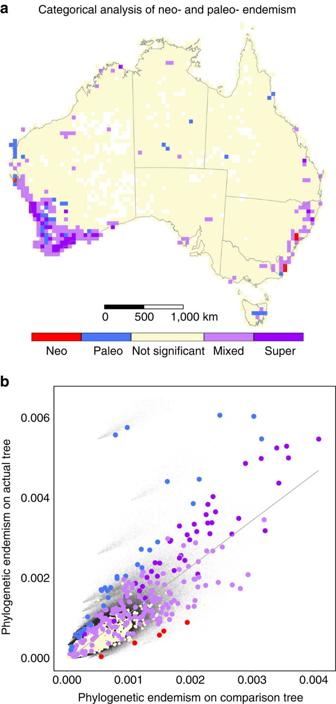Figure 3: CANAPE, a two-step procedure described in text. (a) Map of centres of endemism discovered. White cells contain no records; beige cells are not significant. The red values indicate grid cells that contain significantly lower RPE than expected given random sampling of the same number of species from a null tree, termed ‘centres of neo-endemism’. The blue values indicate grid cells that contain significantly higher RPE than expected, termed ‘centres of paleo-endemism’. The purple values indicate grid cells that are a mix of neo-endemism and paleo-endemism; the most highly significant of which (darker purple) are termed ‘centres of super-endemism’. (b) Bivariate plot showing the relationship between the numerator (yaxis) and denominator (xaxis) of RPE, applied following the two-step CANAPE procedure described in text, for comparison witha. The grey points in the background are results of the randomization, the beige points are actual values for grid cells that are not significant, the red points are actual values for grid cells that are interpreted as significantly dominated by neo-endemism, the blue points are actual values for grid cells that are interpreted as significantly dominated by paleo-endemism, and the purple points are actual values for grid cells significant for both they-axis andx-axis variables separately, the most highly significant of which (darker purple) are termed ‘centres of super-endemicity’. Full size image Figure 3a shows the results of the two-step CANAPE described in the Methods, while Fig. 3b shows a bivariate plot comparing the numerator and denominator of RPE, used in CANAPE, to help understand the classification of centres of endemism shown in Fig. 3a . Areas with grid cells dominated by paleo-endemism include southwestern Australia, the Gascoyne Region, central Australia, wet tropic sites in Queensland and Tasmania. Grid cells dominated by neo-endemism are restricted to the coast of New South Wales. Areas of mixed endemism are mainly in southwestern Australia and along the southeast coast, with super-endemic sites largely confined to the Southwest. Figure 3: CANAPE, a two-step procedure described in text. ( a ) Map of centres of endemism discovered. White cells contain no records; beige cells are not significant. The red values indicate grid cells that contain significantly lower RPE than expected given random sampling of the same number of species from a null tree, termed ‘centres of neo-endemism’. The blue values indicate grid cells that contain significantly higher RPE than expected, termed ‘centres of paleo-endemism’. The purple values indicate grid cells that are a mix of neo-endemism and paleo-endemism; the most highly significant of which (darker purple) are termed ‘centres of super-endemism’. ( b ) Bivariate plot showing the relationship between the numerator ( y axis) and denominator ( x axis) of RPE, applied following the two-step CANAPE procedure described in text, for comparison with a . The grey points in the background are results of the randomization, the beige points are actual values for grid cells that are not significant, the red points are actual values for grid cells that are interpreted as significantly dominated by neo-endemism, the blue points are actual values for grid cells that are interpreted as significantly dominated by paleo-endemism, and the purple points are actual values for grid cells significant for both the y -axis and x -axis variables separately, the most highly significant of which (darker purple) are termed ‘centres of super-endemicity’. Full size image Identifying and comparing areas of endemism Two hundred and forty-six grid cells of significantly high endemism were identified from the results of the CANAPE test. The cluster analysis using PD-dissimilarity ( Fig. 4 ) revealed that these grid cells tend to cluster geographically. The southeast (blue), southern South Australia (turquoise) and many central locations (brown) are more similar in terms of the parts of the phylogenetic tree they share as compared with the southwest (shades of green) and western central areas (shades of red and purple). Interestingly, the greatest diversity of phylo-clusters is present in central-west Western Australia, and there is a major biogeographic break observable between the southwest and areas immediately north in the Wheat Belt and central Western Australia coast. 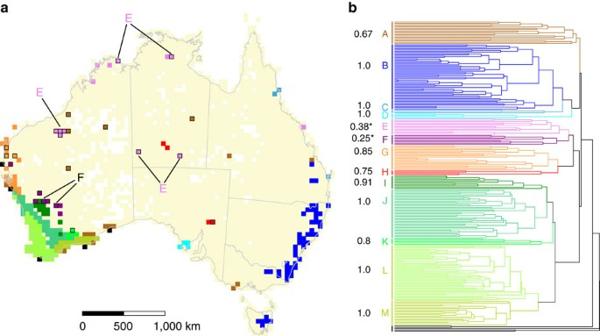Figure 4: Map (a) and cluster analysis (b) showing phylogenetic similarity relationships among centres of endemism for AustralianAcacia. The cluster analysis used PD-dissimilarity and a phylo-jaccard metric with link-average linkage. Areas that cluster closely, indicating that they share many branches of their phylogenetic subtrees, are shown in the same colour and lettered for reference in the text. The number given by each letter is the proportion of grid cells in that cluster that are at least partly covered by currently protected areas; E and F, the most poorly protected, are marked with an asterisk. The arrows on the map point to the grid cells in clusters E and F that lie completely outside of protected areas and are thus of highest conservation concern. Figure 4: Map (a) and cluster analysis (b) showing phylogenetic similarity relationships among centres of endemism for Australian Acacia . The cluster analysis used PD-dissimilarity and a phylo-jaccard metric with link-average linkage. Areas that cluster closely, indicating that they share many branches of their phylogenetic subtrees, are shown in the same colour and lettered for reference in the text. The number given by each letter is the proportion of grid cells in that cluster that are at least partly covered by currently protected areas; E and F, the most poorly protected, are marked with an asterisk. The arrows on the map point to the grid cells in clusters E and F that lie completely outside of protected areas and are thus of highest conservation concern. Full size image Investigating the phylogenetic patterns of biodiversity and endemism adds significantly to the traditional approach that considers species diversity alone. For example, 13 out of 21 previously recognized centres of raw species endemism in Acacia (that is, comparable to the measure shown in Fig. 1b ) are located in the southeastern and southwestern temperate regions of Australia [26] . Many of the centres of PE found in this study are located in the same regions, but add new localities previously unidentified by the traditional species-based metrics ( Fig. 3a ). These results provide critical information that can guide conservation planning because they locate biodiversity centres in terms of evolutionary history and potential refugia. The null hypothesis for testing the phylogenetic measures employed here requires a tree, since PD and PE are only defined given a tree. One tree that can be used is the actual tree, and indeed the basic hypothesis test of PD and PE we applied (shown in Fig. 2a,c ) simply compares the observed value with what one would expect if the same number of taxa were randomly drawn from the actual tree, similar to the relative phylogenetic diversity (PD rel ) measure of Davies et al. [27] This allows one to infer whether the measure is significantly high or low for a given number of terminal taxa drawn from that tree, but this test is entirely dependent on the particular tree at hand, and not comparable to other studies underlain by a different tree. One could attempt to generalize solely based on the number of terminal taxa present, but that would not be a sound reasoning without basing the expectation for PD and PE on a generalizable comparison tree giving relationships among the terminal taxa. Therefore, to have a more general, useful and completely phylogenetic null model, we developed two derived metrics that are new to this study, RPD and RPE, both ratios that compare the PD or PE observed on the actual tree in the numerator to that observed on a comparison tree in the denominator. Several comparison tree topologies were explored in this study, but only one was employed for the analyses presented here, as it represents the most generalized null model for our purposes. This comparison tree gives the expectation for PD and PE if all branches on the actual tree topology (interior and exterior) were equal in terms of branch length. This tree is equivalent to one commonly used early approach to measurement of PD that counted nodes on a tree [9] , [11] , and is equivalent to a punctuational model of evolution. The hypothesis test of RPD or RPE tells one how much observed PD or PE differs from that null expectation, for example, asking ‘is PD significantly high or low compared to what I would expect with that number of terminal taxa randomly selected from my tree if all its branches were equal in length?’ The expectation of the ratio is 1, and significant departure from the expected allows us determine if there is an over-representation of long branches or short branches on the actual tree, an important innovation that is useful for addressing several key biological questions, as detailed below. Significantly high RPD indicates an area where there is an over-representation of long branches. This could have several alternative explanations. One possibility is historical biogeography: the area is refugial, containing relicts from past climate change [28] . Another possibility is ecology: the result of competition that prohibits close relatives from co-occurring in the same communities (that is, phylogenetic overdispersion [8] ). Separating these two possible causes would be assisted by mapping ecologically significant variables to the tree. Significantly low RPD indicates an area where there is an over-representation of short branches. This pattern also could have alternative explanations, including evolutionary: the area is a place of recent divergence of lineages. Another possibility is ecological: the result of habitat filtering based on phylogenetically conserved traits that result in close relatives co-occurring in the same communities (that is, phylogenetic clustering [8] ). Adding ages on branches would help separate these explanations as would mapping ecologically significant variables to the tree. This comparison tree is particularly useful for the purpose of distinguishing centres of neo-endemism and paleo-endemism. Since PE is simply the PD of a range-weighted tree (that is, where each branch has been divided by its range size), then when RPE is significantly greater than 1 it must mean there is an over-representation of rare long branches and when it is significantly less than 1 it must mean there is an over-representation of rare short branches. This is because rare long branches, whether terminal branches or deeper, in the actual tree are longer than the null expectation and vice-versa for rare short branches. However, since RPE is a ratio, if the purpose is identifying centres of significant endemism, it is important to realize that spurious conclusions are possible when interpreting the significance of RPE. It is possible to have a significantly high or low RPE ratio when both the numerator and denominator are quite small, and hence when there is not a significant amount of endemism present. Thus we realized that a two-step process is necessary for finding areas of significant PE; we need to first establish that there is a significant amount of endemism in a grid cell, then use the RPE ratio to parse the significant centres of endemism into those dominated by rare long branches (paleo-endemism), those dominated by rare short branches (neo-endemism) and those with rare branches of mixed lengths. This is the two-step CANAPE test described in the Methods. By comparing Fig. 2d with Fig. 3a , it is possible to see the need for the two-step approach: Fig. 2d shows some grid cells that are significantly high or low in RPE that are not actually centres of PE and thus are not significant in Fig. 3a . The scatter plot in Fig. 3b helps to show what is going on: the randomized values are grey, and most are clustered in the lower left corner along with the nonsignificant actual values (beige coloured). Of the significant actual values, the centres of paleo-endemism (blue) occupy space in the upper left of the distribution, where PE on the actual tree is larger than PE expected on the comparison tree (indicating the rare branches must be longer than expected), while the centres of neo-endemism (red) occupy space in the lower right of the distribution, where PE on the actual tree is less than PE expected on the comparison tree (indicating the rare branches must be shorter than expected). The centres of mixed endemism tend to occur in the upper right of the distribution, with the highly significant values (here termed super-endemism) in the far upper right. In this way, CANAPE is able to distinguish different types of centres of endemism, and can thus give insights into different evolutionary and ecological processes that may be responsible for these patterns. The centres of paleo-endemism indicate places where there are over-representation of long branches that are rare across the landscape. This pattern seems to be a clear indication of refugial areas where clades that are present may have suffered high extinction and range contraction in past eras. Note that there could be centres of paleo-endemism superimposed geographically in an area that is caused by climatic or geological events at different times in the earth’s history. This would be indicated if the rare long branches of an area group into two or more different age categories in a dated phylogeny. We identified several areas of paleo-endemism in Acacia using the CANAPE test ( Fig. 3a ). These areas include the wet tropics in northern Queensland, central alpine areas of Tasmania, southwest Western Australia, the Gascoyne region in Western Australia and scattered areas in the arid centre of the continent. The centres of neo-endemism indicate an area where there is an over-representation of short branches that are rare on the landscape. This could, for example, indicate a place where peripheral isolates tend to diversify, thus enabling studies of speciation. We identified only a few areas of neo-endemism in Acacia using the CANAPE test in southeastern Australian including the Greater Sydney Basin. Centres of a third type of endemism were identified by CANAPE in the southwest and southeast ( Fig. 3a ), complex centres containing a mixture of both paleo-endemism and neo-endemism. The most highly significant of these sites we here term ‘super-endemic’ sites—such sites are mostly restricted to the mega-diverse southwest. The two main areas of super-endemism are north of Perth in the Wheat belt area and along the Albany coast. The cluster analysis, using PD-dissimilarity to compare only those grid cells that were determined to be significant centres of endemism ( Fig. 4 ), gives insights into relationships among them based on shared branches of the phylogeny. The temperate region of Australia is subdivided into mainly western and mainly eastern clusters. The Southwestern Australian Floristic Region [29] is recognized as one of the world’s biodiversity hotspots. We found a cluster specific to that zone (I, J, K, L and M in Fig. 4 ); there is interesting geographic substructure in this region with a distinctive SW–NE gradient. These gradients are well documented in the literature and mainly reflect the high rainfall zone on the western regions, a semi-arid transitional rainfall zone towards the north east and a southeastern zone with relatively high rainfall [29] . Clusters E and F consist of sites scattered in the interior and north. Cluster H groups sites in the Eremaean biome in the centre of the continent and South Australia, while cluster A groups scattered sites in the centre of the continent and the southern coast of Victoria and Western Australia. Cluster D groups a distinctive set of sites on the southern coast of South Australia. The Southeast temperate biome (including Tasmania), contains areas of mountains with a combination of tropical, subtropical and Mediterranean climates; it is represented by cluster B. Wet tropical sites in coastal northern Queensland (cluster C) are quite distinct, but group with cluster B rather than with the sites in the northern tropical Monsoonal biome (cluster E), which includes all of the northern regions from the Kimberley to Cape York Peninsula. The Gascoyne cluster (cluster G) is located on the western side of the Eremaean biome in an area of topographical complexity and interestingly groups with the monsoonal and central Western Australia clusters E and F rather than the nearby southwestern cluster (I, J, K, L and M), marking a major biogeographic break. Conservation prioritization can be evaluated from Figs 3a and 4 . For example, the three most important large areas of paleo-endemism to conserve in terms of complementarity with each other would be southwest Western Australia, the Gascoyne region and Tasmania. Reserves located in central-west Western Australia would capture more PD than any others. By overlaying our results with the current protected areas database [30] we found 25 cells that do not intersect with any currently protected areas. These cells fell into seven of the clusters (A, E, F, G, H, I and K) and are indicated with black borders on the map in Fig. 4 . The clusters with the poorest current protection are E and F, their unprotected grid cells are pointed out in Fig. 4 . Much future work is needed for the continent of Australia (and elsewhere) to add comparable analyses of PD and PE in other groups with different phylogenetic time-depths and biological attributes. The methods proposed here allow, for the first time, a quantitative distinction between centres of neo-endemism and centres of paleo-endemism, and enable meta-analyses across groups to identify general patterns in the biota for ecological and evolutionary explanation and for overall conservation assessment. These methods are valuable additions to the conservation decision-making process; reserve design can be guided by assessment of phylogeny rather than species counts alone and can identify complementary areas of biodiversity [12] that have unique evolutionary histories and traits in need of conservation. Assembly of geographic data We extracted all Acacia records from the Australia’s Virtual Herbarium database [31] , totalling 218,388 records. These were corrected as outlined in González-Orozco et al. [26] To ensure a standard taxonomy in the analyses, we only used species names accepted by the Australian Plant Census [32] . Varieties and subspecies were included at the species level. A total of 171,758 records remained following the correction process, comprising the 1,020 species of Acacia occurring in Australia. A data subset, containing 132,295 records, was generated that contained the data for the 508 species, which are sampled in the phylogenetic analysis. This data set is available from the Dryad digital repository: http://doi.org/10.5061/dryad.dv4qk . Assembly of molecular data The sampling consisted of 510 taxa, representing single specimens of 508 Acacia species, and two outgroup taxa, Parachidendron pruionsum and Paraserianthes lophantha subsp. lophantha , that were selected based on results of previous studies [33] , [34] , [35] , [36] , [37] . Each Acacia species in the sample set was chosen from a larger set of 1,152 sequenced samples of the same 508 species in the following way. In the majority of cases, multiple specimens of a single species were monophyletic and the specimen with the best DNA sequence coverage of the six DNA loci was used to represent that species. In the case that multiple specimens representing a species were polyphyletic, the representative specimen was chosen by (1) belonging to the largest clade of specimens for that species and (2) by reference to the Flora of Australia [23] . DNA was extracted from fresh leaf samples that were collected either in the field or from cultivated plants of known provenance, and where no other material was available, from herbarium specimens. Six regions were amplified and sequenced, which included four plastid: psb A -trn H intergenic spacer, trn L-F intron and intergenic spacer, rpl 32-trnL intergenic spacer, and a portion of the mat K intron, and two nuclear: ETS and ITS. Details of the procedures can be found in Miller et al. [38] All DNA sequences are deposited in Genbank; accession codes for sequences newly generated for this study are provided in the Accession codes section below (see also Supplementary Table 1 ). Phylogenetic analyses Contiguous sequences were edited using Sequencher v.3.0 (Gene Codes Corporation) and manually aligned in Se-Al [39] . Sequence alignments and Nexus formatted files are available from the authors upon request and lodged in TreeBase (ID 13659). Any uncertain base positions, generally located close to priming sites, and highly variable regions with uncertain sequence homology were excluded from phylogenetic analysis. A maximum likelihood analysis was performed on the 4,044-bp data set in the CIPRES Portal ( www.phylo.org ) using the RAxML HPC BlackBox tool with a partition model set for each locus. The resulting bipartition tree was saved and FigTree [40] was used to view and generate a Nexus format tree suitable for the biodiversity analyses. Basic biodiversity analyses We projected the locality data using Australian Albers equal area EPSG:3577 (ref. 41 ) and used the program Biodiverse (version 0.17 (ref. 42 )) to calculate four standard indices: SR, WE, PD and PE for equal-area square grid cells (50 × 50 km) covering the continent of Australia including Tasmania (3,037 grid cells in all). Development of null hypotheses Raw values of PD and PE are not highly informative; it is necessary to know whether the observed values are higher or lower than one expects given a null model. For example, the magnitude of PD and PE are clearly affected by the number of terminal taxa present. Therefore, the significance of PD and PE can be tested in one way by comparing the actual value for a grid cell with the value for many random selections of the same number of terminal taxa from the same tree [27] , and this was done in the present study. We also calculated for each grid cell two derived metrics that are new to this study and have been added as extensions of the Biodiverse package: RPD and RPE. Both of these indices are ratios that compare the PD and PE observed on the actual tree in the numerator to that observed on a comparison tree in the denominator. To make them easily comparable between analyses, the trees in both the numerator and the denominator are scaled such that branch lengths are calculated as a fraction of the total tree length. The comparison tree retains the actual tree topology but makes all branches of equal length. Thus, RPD is PD measured on the actual tree divided by PD measured on the comparison tree, while RPE is PE measured on the actual tree divided by PE measured on the comparison tree. In combination with the randomization test (below), this lets us examine the extent to which differential branch lengths matter to the patterns of PD and PE observed, which is important to our goals. Randomization tests The statistical significance of PD, PE, RPD and RPE were assessed using a randomization with a null model that retained some of the structural features of the data (using the ‘rand_structured’ option in Biodiverse). In this model, species occurrences in grid cells are randomly reassigned to grid cells without replacement, thus keeping constant both the total number of grid cells for each species and the SR of each grid cell [17] . We ran 999 trials of the randomization null model, calculating PD, PE, RPD and RPE for each trial. These values formed a null distribution for each grid cell for use in non-parametric tests of the significance of observed values. For all variables, a two-tailed test was applied as both indices can have values significantly higher or significantly lower than the null. If the observed value fell into the highest 2.5% of the distribution for that grid cell it was judged significantly high; if the observed value fell into the lowest 2.5% of the distribution for that grid cell it was judged significantly low. We also observed results using a more conservative 1% confidence level. We used R scripts to generate map visualizations of the results overlaying the coloured raster data with map outlines. Software and links for performing these tests and visualizations has been made publicly available at the Biodiverse website ( http://purl.org/biodiverse ). Identifying areas of endemism To find and distinguish different types of centres of endemism, we followed a two-step process using RPE that we call CANAPE. First, to determine whether a place is a centre of significantly high endemism, a grid cell needs to be significantly high (one-tailed test, α =0.05) in the numerator of RPE, the denominator or both. If (and only if) grid cells pass one of those tests, then they are divided into three meaningful, non-overlapping categories of centres of endemism in this way: if a point is significantly high or low in the RPE ratio (two-tailed test, α =0.05), then it is a centre of paleo-endemism or neo-endemism, respectively; if it is significantly high in both the numerator and the denominator (taken alone), but not significant for RPE, then it is a centre of mixed endemism. The latter category can be interpreted as a centre of endemism having a mix of rare long and rare short branches, so not significantly dominated by either paleo-endemism or neo-endemism. The mixed endemism areas were further subdivided; those grid cells that are significantly high in both the numerator and the denominator at the α =0.01 level are termed super-endemic sites. Comparisons among identified areas of endemism Grid cells that were identified as statistically significant centres of endemism were then compared using PD-dissimilarity as implemented using the ‘phylo_Jaccard’ measure using a weighted average linkage and visualized using cluster analyses in the program Biodiverse [42] . We intersected the 246 cells with The Collaborative Australian Protected Areas Database [30] and identified cells containing protected areas and cells where protected areas were absent. We also compared these centres of endemism to previously defined biomes of Australia [43] to check for correspondence of the biome boundaries with specific clusters. Accession codes: All DNA sequences generated in this study have been deposited in GenBank nucleotide database under accession codes: KC013753 , KC013759 , KC013773 , KC200572 , KC200574 – KC200577 , KC200579 , KC200581 , KC200583 , KC200586 , KC200589 , KC200590 , KC200593 – KC200595 , KC200598 , KC200599 , KC200603 , KC200604 , KC200607 , KC200614 , KC200616 , KC200617 , KC200619 , KC200620 , KC200624 – KC200627 , KC200629 , KC200631 – KC200633 , KC200635 , KC200636 , KC200639 , KC200640 , KC200643 , KC200644 , KC200647 – KC200649 , KC200651 , KC200653 , KC200654 , KC200657 – KC200662 , KC200665 , KC200667 , KC200669 , KC200673 – KC200678 , KC200682 , KC200683 , KC200685 , KC200688 , KC200689 , KC200695 , KC200696 , KC200698 , KC200702 , KC200705 – KC200707 , KC200710 , KC200714 – KC200720 , KC200722 , KC200725 , KC200729 , KC200731 , KC200733 , KC200735 – KC200737 , KC200740 , KC200744 – KC200747 , KC200753 , KC200755 , KC200758 , KC200762 , KC200766 , KC200770 – KC200774 , KC200777 – KC200779 , KC200789 , KC200791 , KC200792 , KC200794 , KC200796 , KC200799 – KC200801 , KC200806 – KC200808 , KC200812 – KC200814 , KC200816 – KC200820 , KC200823 , KC200828 , KC200831 – KC200836 , KC200840 – KC200846 , KC200848 – KC200853 , KC200856 , KC200857 , KC200860 – KC200862 , KC200864 , KC200866 – KC200870 , KC200874 , KC200877 , KC200879 , KC200881 – KC200885 , KC200891 , KC200892 , KC200902 – KC200904 , KC200906 , KC200908 , KC200909 , KC200914 , KC200918 , KC200920 , KC200925 , KC200926 , KC200930 , KC200932 , KC200933 , KC200935 , KC200937 , KC200938 , KC200940 , KC200945 , KC200947 – KC200949 , KC200951 , KC200954 , KC200956 , KC200958 , KC200959 , KC200962 , KC200963 , KC200965 – KC200968 , KC200970 , KC200971 , KC200973 – KC200976 , KC200982 – KC200984 , KC200986 , KC200987 , KC200990 , KC200991 , KC200993 – KC200996 , KC200998 – KC201000 , KC201005 , KC201006 , KC201008 – KC201010 , KC201013 , KC201014 , KC201018 , KC201019 , KC201021 , KC201023 , KC201028 – KC201030 , KC201033 , KC201034 , KC201044 – KC201046 , KC201048 – KC201050 , KC201052 – KC201054 , KC201056 , KC201058 , KC201059 , KC201062 , KC201065 , KC201068 – KC201073 , KC201075 , KC201076 , KC201088 , KC201090 , KC201091 , KC201093 , KC201094 , KC201098 , KC201100 , KC201102 , KC201106 – KC201111 , KC201114 , KC201115 , KC201117 , KC201118 , KC201122 , KC201132 , KC201134 , KC201135 , KC201138 , KC201141 , KC201142 , KC201147 , KC201154 – KC201157 , KC201164 , KC201165 , KC283245 , KC283246 , KC283248 , KC283251 , KC283255 , KC283257 , KC283260 , KC283261 , KC283264 – KC283266 , KC283271 , KC283272 , KC283274 , KC283276 , KC283278 – KC283284 , KC283286 – KC283288 , KC283290 , KC283292 , KC283296 – KC283301 , KC283304 – KC283311 , KC283313 , KC283314 , KC283316 , KC283319 – KC283322 , KC283325 – KC283327 , KC283330 , KC283332 , KC283334 – KC283336 , KC283338 – KC283346 , KC283348 , KC283350 , KC283351 , KC283354 – KC283358 , KC283360 , KC283362 , KC283363 , KC283366 , KC283369 – KC283371 , KC283376 , KC283380 , KC283381 , KC283384 , KC283386 – KC283390 , KC283393 – KC283406 , KC283408 , KC283409 , KC283411 , KC283412 , KC283417 , KC283421 , KC283423 , KC283430 – KC283432 , KC283438 , KC283441 , KC283443 , KC283447 , KC283453 , KC283464 , KC283472 – KC283478 , KC283480 , KC283484 , KC283486 , KC283488 – KC283490 , KC283492 , KC283493 , KC283495 , KC283497 – KC283499 , KC283501 – KC283506 , KC283509 , KC283510 , KC283512 – KC283519 , KC283521 , KC283523 , KC283525 – KC283527 , KC283529 , KC283532 , KC283533 , KC283535 – KC283538 , KC283540 , KC283541 , KC283543 , KC283547 , KC283548 , KC283550 – KC283553 , KC283555 , KC283556 , KC283593 , KC283598 , KC283609 , KC283618 , KC283641 , KC283643 – KC283646 , KC283649 , KC283653 , KC283654 , KC283662 , KC283671 , KC283676 , KC283680 , KC283683 , KC283690 , KC283692 – KC283698 , KC283700 , KC283701 , KC283705 , KC283706 , KC283708 , KC283709 , KC283711 , KC283714 , KC283715 , KC283717 , KC283718 , KC283720 – KC283722 , KC283724 , KC283725 , KC283727 , KC283729 , KC283733 , KC283735 , KC283742 , KC283745 , KC283748 , KC283756 , KC283761 , KC283765 , KC283767 , KC283773 , KC283774 , KC283780 , KC283783 , KC283789 , KC283790 , KC283797 , KC283801 , KC283802 , KC283807 , KC283810 , KC283815 , KC283818 , KC283820 , KC283822 , KC283823 – KC283828 , KC283830 , KC283831 , KC283833 , KC283835 – KC283837 , KC283839 – KC283841 , KC283844 – KC283846 , KC283848 , KC283850 , KC283853 , KC283856 , KC283858 , KC283859 , KC283864 , KC283865 , KC283868 , KC283870 , KC283872 , KC283873 , KC283875 – KC283878 , KC283881 , KC283883 , KC283884 , KC283886 – KC283891 , KC283893 – KC283899 , KC283911 , KC283916 , KC283920 , KC283923 , KC283925 , KC283926 , KC283930 – KC283932 , KC283934 , KC283938 , KC283942 , KC283945 – KC283947 , KC283950 , KC283953 , KC283957 – KC283960 , KC283961 , KC283966 , KC283967 , KC283970 , KC283973 , KC283980 , KC283982 , KC283983 , KC283985 , KC283989 – KC283992 , KC283995 , KC283996 , KC283998 , KC284002 – KC284008 , KC284011 , KC284012 , KC284014 – KC284016 , KC284019 – KC284022 , KC284025 , KC284031 , KC284034 , KC284041 , KC284043 – KC284045 , KC284047 , KC284049 , KC284052 – KC284057 , KC284059 , KC284060 – KC284063 , KC284067 , KC284071 , KC284074 , KC284078 – KC284083 , KC284086 , KC284090 , KC284091 , KC284093 , KC284096 , KC284098 , KC284099 , KC284101 , KC284108 , KC284112 , KC284116 , KC284119 – KC284121 , KC284123 , KC284128 , KC284131 – KC284133 , KC284136 , KC284138 – KC284141 , KC284143 , KC284146 , KC284147 , KC284151 , KC284153 , KC284154 , KC284156 , KC284158 , KC284159 , KC284161 , KC284164 , KC284165 , KC284168 , KC284170 , KC284174 , KC284175 , KC284177 , KC284178 , KC284184 , KC284186 , KC284187 , KC284189 , KC284192 , KC284196 , KC284205 – KC284209 , KC284215 – KC284218 , KC284220 , KC284222 , KC284224 , KC284225 , KC284227 , KC284228 , KC284230 , KC284233 – KC284237 , KC284243 – KC284246 , KC284251 , KC284254 – KC284257 , KC284261 – KC284263 , KC284265 , KC284269 , KC284273 , KC284274 , KC284276 – KC284278 , KC284280 , KC284281 , KC284282 , KC284287 – KC284293 , KC284295 , KC284297 , KC284300 – KC284302 , KC284305 , KC284306 , KC284309 , KC284310 , KC284312 , KC284314 , KC284316 , KC284317 , KC284319 , KC284321 – KC284325 , KC284332 , KC284334 , KC284341 , KC284343 – KC284346 , KC284349 , KC284350 – KC284353 , KC284355 – KC284358 , KC284360 , KC284362 , KC284364 , KC284365 , KC284371 , KC284375 , KC284377 , KC284380 , KC284385 – KC284387 , KC284390 , KC284394 , KC284397 , KC284398 , KC284400 , KC284404 , KC284407 , KC284409 , KC284416 , KC284423 , KC284424 , KC284429 , KC284435 , KC284437 , KC284438 , KC284441 , KC284446 , KC284449 , KC284451 , KC284453 , KC284456 – KC284458 , KC284461 , KC284462 , KC284465 , KC284466 , KC284469 , KC284470 , KC284473 , KC284476 , KC284481 , KC284483 , KC284488 , KC284489 , KC284494 , KC284496 – KC284500 , KC284502 , KC284508 , KC284511 , KC284513 – KC284517 , KC284519 , KC284524 , KC284525 , KC284529 , KC284530 , KC284531 , KC284533 – KC284535 , KC284538 , KC284540 , KC284548 , KC284550 , KC284552 , KC284554 , KC284555 , KC284557 , KC284560 – KC284562 , KC284566 , KC284567 , KC284569 – KC284571 , KC284573 , KC284575 , KC284577 , KC284580 , KC284587 , KC284592 , KC284595 – KC284600 , KC284602 , KC284604 , KC284608 , KC284612 – KC284616 , KC284620 – KC284622 , KC284628 , KC284629 , KC284631 , KC284638 , KC284641 , KC284642 , KC284644 , KC284645 , KC284647 , KC284650 , KC284651 , KC284655 , KC284656 , KC284658 , KC284660 , KC284664 , KC284665 , KC284667 – KC284669 , KC284671 , KC284673 , KC284676 , KC284677 , KC284679 – KC284682 , KC284685 , KC284688 , KC284690 , KC284696 , KC284698 , KC421182 , KC421185 , KC421186 , KC421189 – KC421192 , KC421198 , KC421201 , KC421202 , KC421206 , KC421208 – KC421216 , KC421218 – KC421220 , KC421222 , KC421224 , KC421228 – KC421234 , KC421237 – KC421242 , KC421244 , KC421247 , KC421249 , KC421250 , KC421254 , KC421256 – KC421259 , KC421261 , KC421263 , KC421265 , KC421267 – KC421276 , KC421278 , KC421279 , KC421281 , KC421282 , KC421286 – KC421293 , KC421295 , KC421297 , KC421298 , KC421302 , KC421305 , KC421307 – KC421310 , KC421317 , KC421320 , KC421322 , KC421327 , KC421332 , KC421333 , KC421335 , KC421339 , KC421340 , KC421348 – KC421353 , KC421355 – KC421361 , KC421363 , KC421365 , KC421366 , KC421368 , KC421373 , KC421374 , KC421376 , KC421381 – KC421383 , KC421390 , KC421393 , KC421394 , KC421397 – KC421399 , KC421403 , KC421404 , KC421406 – KC421409 , KC421411 , KC421414 , KC421416 – KC421420 , KC421423 – KC421427 , KC421429 – KC421431 , KC421433 – KC421436 , KC421439 , KC421440 , KC421442 – KC421448 , KC421450 , KC421453 – KC421457 , KC421459 , KC421462 , KC421463 , KC421465 – KC421468 , KC421470 , KC421471 , KC421473 , KC421477 , KC421478 , KC421480 – KC421482 , KC421484 , KC421487 , KC421532 , KC421553 , KC421570 , KC421572 – KC421575 , KC421578 , KC421581 , KC421583 , KC421591 , KC421597 , KC421602 , KC421607 , KC421612 , KC421620 , KC421622 – KC421625 , KC421627 , KC421628 , KC421701 , KC421704 , KC421705 , KC421708 – KC421710 , KC421713 – KC421715 , KC421717 , KC421720 – KC421726 , KC421728 – KC421730 , KC421732 , KC421733 , KC421736 , KC421737 , KC421742 , KC421744 , KC421751 , KC421756 , KC421758 , KC421766 , KC421776 – KC421779 , KC421782 – KC421784 , KC421788 , KC421789 , KC421791 , KC421792 , KC421795 – KC421797 , KC421799 , KC421800 , KC421802 , KC421804 , KC421809 – KC421811 , KC421819 , KC421825 , KC421826 , KC421831 , KC421836 , KC421840 , KC421843 , KC421845 , KC421847 – KC421853 , KC421856 , KC421857 , KC421859 , KC421861 – KC421863 , KC421865 – KC421867 , KC421870 , KC421870 – KC421872 , KC421871 , KC421872 , KC421875 , KC421877 , KC421879 , KC421882 , KC421885 , KC421887 , KC421888 , KC421893 , KC421895 , KC421896 , KC421900 , KC421901 , KC421903 , KC421904 , KC421906 – KC421908 , KC421910 , KC421911 , KC421913 , KC421915 , KC421916 , KC421918 – KC421920 , KC421922 , KC421923 , KC421924 , KC421927 – KC421929 , KC421932 – KC421934 , KC421949 , KC421956 , KC421960 , KC421964 , KC595994 – KC595998 , KC598181 – KC598193 , KC610557 – KC610566 , KC796097 – KC796100 , KC796103 , KC796104 , KC796106 – KC796134 , KC796136 – KC796159 , KC796161 – KC796164 , KC796170 – KC796177 , KC796179 – KC796182 , KC796184 – KC796200 , KC796202 – KC796225 , KC796228 – KC796230 , KC807392 , KC955264 , KC955265 , KC955269 , KC955301 , KC955784 , KC955885 , KC956526 , KC957123 , KC957129 , KC957130 , KC957134 , KC957583 , KC957587 , KC957588 , KC957591 , KC957593 , KC957598 , KC957601 , KC957610 , KC957619 , KC957624 , KC957625 , KC957629 , KC957638 , KC957640 , KC957641 , KC957644 , KC957645 , KC957647 , KC957650 , KC957655 – KC957657 , KC957660 – KC957662 , KC957664 , KC957667 – KC957673 , KC957676 – KC957678 , KC957680 , KC957681 , KC957683 , KC957686 , KC957687 , KC957692 , KC957695 , KC957699 , KC957704 , KC957706 , KC957708 , KC957716 , KC957720 , KC957724 , KC957726 , KC957731 , KC957733 , KC957741 , KC957744 , KC957751 , KC957756 , KC957758 , KC957760 , KC957761 , KC957764 , KC957765 , KC957768 – KC957770 , KC957772 , KC957773 , KC957776 , KC957778 , KC957781 – KC957783 , KC957786 , KC957787 , KC957791 , KC957792 , KC957795 , KC957796 , KC957799 – KC957801 , KC957806 – KC957808 , KC957810 , KC957812 , KC957818 – KC957820 , KC957829 , KC957835 , KC957836 , KC957840 , KC957845 , KC957850 , KC957853 , KC957855 – KC957862 , KC957865 , KC957866 , KC957868 , KC957870 – KC957872 , KC957874 – KC957876 , KC957879 , KC957880 , KC957883 , KC957885 , KC957887 , KC957890 , KC957893 , KC957894 , KC957897 , KC957899 , KC957900 , KC957904 , KC957906 , KC957908 , KC957909 , KC957911 – KC957913 , KC957915 , KC957916 , KC957918 , KC957919 , KC957921 , KC957922 , KC957925 , KC957926 , KC957931 , KC957933 – KC957936 , KC957951 , KC957959 , KC957967 , KC957971 – KC957973 , KC957976 , KC957979 , KC957981 , KC957985 , KC957987 – KC957990 , KC957993 , KC957995 , KC957997 , KC958000 , KC958001 , KC958003 – KC958005 , KC958007 , KC958008 , KC958012 , KC958014 – KC958018 , KC958020 , KC958021 , KC958023 – KC958027 , KC958029 , KC958033 , KC958035 , KC958036 , KC958039 , KC958041 , KC958044 , KC958047 – KC958050 , KC958051 , KC958054 , KC958056 , KC958059 , KC958062 , KC958066 , KC958067 , KC958069 , KC958073 , KC958077 – KC958083 , KC958085 , KC958088 – KC958092 , KC958094 , KC958098 , KC958105 , KC958108 , KC958111 , KC958115 – KC958117 , KC958122 , KC958123 , KC958127 , KC958128 , KC958137 – KC958141 , KC958144 , KC958145 , KC958147 – KC958151 , KC958154 , KC958157 , KC958159 – KC958161 , KC958165 , KC958167 , KC958175 – KC958177 , KC958185 , KC958188 , KC958191 – KC958194 , KC958200 , KC958201 , KC958203 , KC958205 , KC958208 , KC958209 , KC958213 , KC958216 , KC958219 , KC958221 , KC958225 , KC958228 , KC958235 , KC958242 , KC958249 , KC958260 , KC958262 , KC958263 , KC958265 – KC958267 , KC958271 , KC958277 – KC958279 , KC958281 – KC958283 , KC958285 , KC958289 , KC958291 , KC958294 , KC958295 , KC958298 – KC958300 , KC958302 – KC958305 , KC958308 , KC958310 , KC958312 , KC958313 , KC958315 – KC958321 , KC958323 , KC958325 , KC958327 , KC958328 , KC958330 , KC958331 , KC958336 , KC958338 , KC958339 , KC958341 – KC958343 , KC958345 , KC958346 , KC958348 , KC958352 – KC958354 , KC958355 , KC958357 , KC958358 , KC958360 , KC958364 , KC958434 , KF048238 , KF048562 , KF048566 – KF048569 , KF048571 , KF048587 , KF048588 , KF048593 , KF048597 , KF048598 , KF048600 , KF048602 , KF048604 , KF048605 , KF048607 , KF048609 , KF048610 , KF048612 – KF048614 , KF048616 – KF048619 , KF048625 , KF048628 , KF048629 , KF048632 , KF048635 , KF048637 , KF048643 , KF048648 , KF048652 , KF048654 , KF048661 , KF048663 , KF048665 , KF048666 , KF048670 , KF048672 , KF048676 – KF048679 , KF048681 , KF048682 , KF048685 , KF048693 , KF048759 , KF048760 – KF048762 , KF048780 – KF048782 , KF048784 – KF048786 , KF048789 , KF048791 , KF048792 , KF048794 – KF048797 , KF048803 , KF048824 , KF048825 – KF048828 How to cite this article: Mishler, B. D. et al. Phylogenetic measures of biodiversity and neo- and paleo-endemism in Australian Acacia . Nat. Commun. 5:4473 doi: 10.1038/ncomms5473 (2014).